Multinuclear nanoliter one-dimensional and two-dimensional NMR spectroscopy with a single non-resonant microcoil Nuclear magnetic resonance (NMR) spectroscopy is a powerful analytical technique, but its low sensitivity and highly sophisticated, costly, equipment severely constrain more widespread applications. Here we show that a non-resonant planar transceiver microcoil integrated in a microfluidic chip (detection volume 25 nl) can detect different nuclides in the full broad-band range of Larmor frequencies (at 9.4 T from 61 to 400 MHz). Routine one-dimensional (1D) and two-dimensional (2D), homo- and heteronuclear experiments can be carried out using the broad-band coil set-up. Noteworthy, heteronuclear 2D experiments can be performed in a straightforward manner on virtually any combination of nuclides (from classical 1 H– 13 C to more exotic combinations like 19 F– 31 P) both in coupled and decoupled mode. Importantly, the concept of a non-resonant system provides magnetic field-independent NMR probes; moreover, the small-volume alleviates problems related to field inhomogeneity, making the broad-band coil an attractive option for, for example, portable and table-top NMR systems. Nuclear magnetic resonance (NMR) spectroscopy is one of the most versatile and powerful analytical tools used in chemistry, physics, biology and medicine. However, the low sensitivity of NMR spectroscopy severely constrains its applications, particularly for mass- and volume-limited samples. Methodologies to enhance the NMR sensitivity comprise expensive and technologically demanding solutions such as ultra-high magnetic fields [1] , cryogenically cooled probes [2] and dynamic nuclear polarization schemes [3] , [4] , or more exotic alternative detection schemes like optical [5] , or remote detection [6] , or travelling wave NMR. [7] Investigation of mass-limited samples can also benefit from the reduction of the sample volume in miniaturized coils, since the amplitude of the NMR signal is optimal when the sizes of the coil and sample match [8] , [9] , [10] . Microcoils with different geometries have proven to be a successful sensitivity enhancement strategy for mass-limited samples [11] , [12] , [13] , [14] , [15] , [16] , although their use remains restricted to date mainly to 1D 1 H-NMR spectroscopy. For heteronuclear and multidimensional NMR experiments, sophisticated and complex electronic circuitry is required [17] , [18] , which limits the more widespread application and implementation of (microcoil) NMR spectroscopy. A classical NMR front end consists of a transmit/receive coil enveloping the sample and a tuning/matching circuit driven through a Z 0 (usually 50 Ω) coaxial cable [19] , [20] . For multi-(frequency) channel probes, this implies multiple coils and/or multi-dip tuning circuits, making the probes very complex. Using non-tuned coils for NMR spectroscopy has been considered in the 60s of last century [21] , [22] ; however, it has remained unexploited in the following decades of developments of ever higher field spectrometers. During the last decade, the ‘non-resonant’ NMR concept has been picked-up again, and shown useful for low-frequency and/or low-resolution NMR applications, already corroborating the validity of this approach [23] , [24] , [25] , [26] . However, none of these report on high-resolution high-field applications, and advanced homo- and heteronuclear two-dimensional (2D) NMR applications of non-tuned coils. Here we present the use of a single transmitter-receiver microcoil in an unconventional simple non-resonant radio frequency (RF) circuit, which allows observation of all NMR-active nuclides with Larmor frequencies from 61 ( 2 H) to 400 ( 1 H) MHz in a 9.4 T system. This most simple set-up allows homo- and heteronuclear, one- and multidimensional NMR experiments to be carried out using one microcoil front end with an excellent mass sensitivity. Heteronuclear 1D NMR experiments We have designed a Broad-Band Coil (BBC) microfluidic NMR chip with a 25 nl detection volume and an integrated planar spiral single transceiver coil directly coupled to a coaxial cable, i.e., without any tuning or matching capacitors ( Fig. 1a–c ; for details on design and fabrication, see Methods and Supplementary Fig. 1 ), which performs well over the full broad RF band relevant for NMR at 9.4 T. To demonstrate the broad-band character of the BBC set-up, spectra of seven different nuclides present in the same sample were sequentially recorded in the 400–61 MHz frequency range ( Fig. 2 ). The normalized 1 H molar sensitivity of the non-tuned BBC probe was of 6,546 signal-to-noise ratio (SNR)·μmol −1 s −1/2 , which is four times higher than the value reported for a 620 nl 1 H-tuned microsolenoid probe and ~50 times higher than the one reported for a 5-mm commercial probe (see the Methods section for calculations) [8] . Moreover, one BBC probe can perform experiments for which normally dedicated and optimized separate probes are used; furthermore, one BBC probe can be used at different magnetic field spectrometers, while normal probes are only functional at a specific magnetic field strength (see Supplementary Note 1 ). This counter-intuitive paradigm shift works because: (i) A spiral coil has broad-band characteristics, with its impedance remaining close to the DC value from 0 MHz up to 400 MHz. (ii) The current passed from an RF source through a coaxial cable into a resistor R remains finite even when R tends to zero, despite the fact that the transmitted power also tends to zero due to power reflection. (iii) The capability of the RF pulse to produce the oscillating magnetic field B 1 depends upon the transmitted current and not, as usually stated, the transmitted power . B 1 is in fact proportional to the current and inversely proportional to the sample-to-coil distance [27] . The current passed through the unmatched BBC set-up is sufficient to produce a very usable B 1 field in the sample across the full RF range. Once a reasonable value of B 1 is reached, the same set-up has also good detection efficiency thanks to the reciprocity theorem [28] and to the fact that during signal reception a low-impedance coil can easily drive a 50 Ω coax and load (the preamplifier). 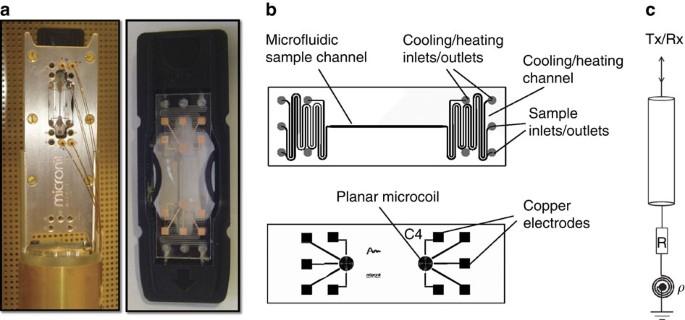Figure 1: Multipurpose NMR chip with two detection areas. (a) photograph of the NMR probe set-up (left) and microfluidic 1.5 × 4.5 cm NMR chip (BBC) inside slider (right). (b) Schematics of the chip with top-side-view (centre), front-view with fluidic channels (top) and back-view with copper electrodes and coil (bottom). (c) RF circuit of the BBC: a microcoil having a DC resistanceρin series with an optional variable resistor (R). SeeSupplementary Informationfor further details of the chip and coil properties. Tx, transmitter. Rx, receiver. Figure 1: Multipurpose NMR chip with two detection areas. ( a ) photograph of the NMR probe set-up (left) and microfluidic 1.5 × 4.5 cm NMR chip (BBC) inside slider (right). ( b ) Schematics of the chip with top-side-view (centre), front-view with fluidic channels (top) and back-view with copper electrodes and coil (bottom). ( c ) RF circuit of the BBC: a microcoil having a DC resistance ρ in series with an optional variable resistor ( R ). See Supplementary Information for further details of the chip and coil properties. Tx, transmitter. Rx, receiver. 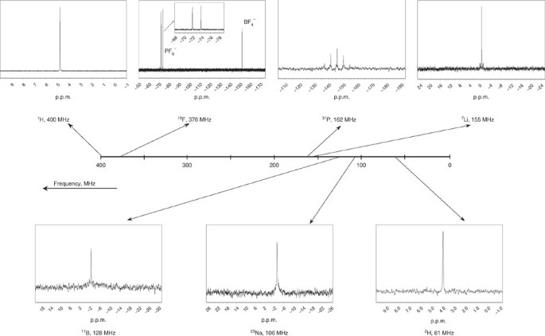Figure 2: Full broad-band 1D NMR detection of seven different nuclides. A 25 nl 50/50% H2O/D2O sample containing 25 nmol of LiPF6and NaBF4reveals:1H (1 scan, 1 s),19F (1 scan, 1 s; the 30 kHz wide19F-NMR spectrum shows the BF4and PF6anion signals, the latter appearing as doublet with characteristic1JPF=710 Hz15),31P (10,000 scans, 10 h),7Li (16 scans, 2 min),11B (64 scans, 2 min),23Na (32 scans, 4 min) and2H (1 scan, 1 s). Differences in SNR between the spectra are due to differences in receptivity of the nuclides and non-optimized 90° pulses at some frequencies. Full size image Figure 2: Full broad-band 1D NMR detection of seven different nuclides. A 25 nl 50/50% H 2 O/D 2 O sample containing 25 nmol of LiPF 6 and NaBF 4 reveals: 1 H (1 scan, 1 s), 19 F (1 scan, 1 s; the 30 kHz wide 19 F-NMR spectrum shows the BF 4 and PF 6 anion signals, the latter appearing as doublet with characteristic 1 J PF =710 Hz [15] ), 31 P (10,000 scans, 10 h), 7 Li (16 scans, 2 min), 11 B (64 scans, 2 min), 23 Na (32 scans, 4 min) and 2 H (1 scan, 1 s). Differences in SNR between the spectra are due to differences in receptivity of the nuclides and non-optimized 90° pulses at some frequencies. Full size image Homo- and heteronuclear 1D and 2D NMR experiments The spectral information of a less-sensitive nuclide, for example, 13 C, is usually recovered from its effect on a more sensitive one, for example, 1 H, provided they are coupled. Such indirect detection experiments are generally carried out employing special probes containing separate coils and/or complex tuning and matching circuits for the individual nuclides to be addressed. The broad-band nature of the BBC enables execution of heteronuclear 1D and 2D NMR experiments, with the single non-tuned NMR microcoil addressing frequencies of different nuclides, separated by hundreds of MHz. 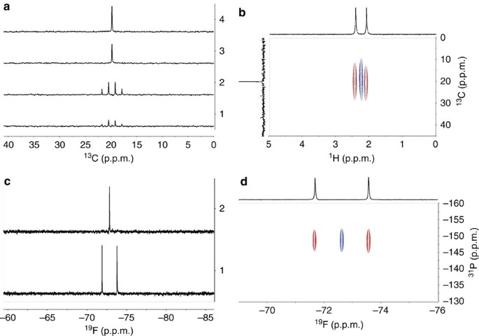Figure 3: Indirect-detection experiments on a single non-resonant microcoil. (a)13C-NMR spectra obtained using different pulse sequence schemes: coupled (1), coupled with nuclear Overhauser effect (NOE) enhancement (2), decoupled without NOE enhancement (3), and decoupled with NOE enhancement (4). (b)1H13C-HSQC spectra. (c) 1D19F-NMR spectra coupled (bottom) and decoupled (top). (d) 2D19F31P-HSQC spectra. The 2D spectra have been acquired in coupled (red) and decoupled (blue) mode. Figure 3 depicts a series of heteronuclear 1D and 2D spectra recorded for a ‘classical’ 1 H– 13 C case (top), and a more exotic combination of nuclides, namely 19 F– 31 P (bottom). Decoupling schemes can be applied during 1D experiment, as shown by 13 C and 19 F-spectra recorded from neat acetic acid-2- 13 C ( Fig. 3a ), respectively, NaPF 6 (1 M solution in H 2 O, Fig. 3c ). In addition, 2D experiments can be performed in coupled and decoupled mode, as illustrated with the 1 H 13 C-HSQC ( Fig. 3b ) and 19 F 31 P-HSQC ( Fig. 3d ) (HSQC, heteronuclear single-quantum coherence) spectra, obtained in just a few minutes representing an additional proof of the striking versatility of the BBC set-up. Figure 3: Indirect-detection experiments on a single non-resonant microcoil. ( a ) 13 C-NMR spectra obtained using different pulse sequence schemes: coupled (1), coupled with nuclear Overhauser effect (NOE) enhancement (2), decoupled without NOE enhancement (3), and decoupled with NOE enhancement (4). ( b ) 1 H 13 C-HSQC spectra. ( c ) 1D 19 F-NMR spectra coupled (bottom) and decoupled (top). ( d ) 2D 19 F 31 P-HSQC spectra. The 2D spectra have been acquired in coupled (red) and decoupled (blue) mode. Full size image Molecular structure analysis 2D homo- and heteronuclear experiments are powerful tools for structure elucidation [29] , and nowadays standard ones on commercial spectrometers include 1 H 1 H-COSY (correlation spectroscopy), 1 H 1 H-NOESY (nuclear Overhauser effect spectroscopy), 1 H 13 C-HSQC and 1 H 13 C-HMBC (heteronuclear multiple-bond correlation). All these experiments were performed using our BBC set-up on 18 μg (100 nmol) ethyl cinnamate ( Fig. 4 ). The resolution in the 2D experiments is comparable to that of spectra obtained with commercial probe set-ups, and they permit full assignment of all 1 H and 13 C signals at natural abundance of the isotopes (for 13 C corresponding to 1 nmol, 40 mM concentration, under the conditions used). The COSY, NOESY, HSQC and HMBC reported here represent the first homo- and heteronuclear 2D experiments performed on a single non-resonant coil. Notably, these experiments were carried out on a quantity of material at least an order of magnitude less than needed on a normal commercial 5 mm probe at the same magnetic field strength (see Supplementary Table 1 ). 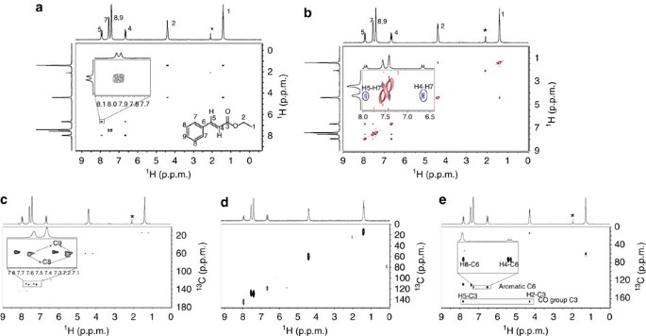Figure 4: High-resolution homo- and heteronuclear 2D NMR. Experiments were performed measuring 18 μg of ethyl cinnamate. COSY (a) and NOESY (b) experiments permit full assignment of all proton signals. The HSQC experiment ((c) coupled, (d) decoupled) allows full characterization of the proton-coupled carbons, including severely overlapping signals. The HMBC (e) experiment further reveals the two quaternary carbon atoms. Residual solvent (toluene) is indicated by an asterisk. Figure 4: High-resolution homo- and heteronuclear 2D NMR. Experiments were performed measuring 18 μg of ethyl cinnamate. COSY ( a ) and NOESY ( b ) experiments permit full assignment of all proton signals. The HSQC experiment (( c ) coupled, ( d ) decoupled) allows full characterization of the proton-coupled carbons, including severely overlapping signals. The HMBC ( e ) experiment further reveals the two quaternary carbon atoms. Residual solvent (toluene) is indicated by an asterisk. Full size image Fluorine NMR spectroscopy The 19 F nuclide represents an attractive alternative to 1 H for both NMR and magnetic resonance imaging applications on different areas such as medicinal chemistry and drug design [30] , polymer chemistry and agrochemicals [31] or contrast agents [32] . On conventional spectrometers, special probes equipped with double-tuned or 19 F-dedicated coils and other specific hardware are required for, and thus preventing a widespread use of, 19 F-NMR spectroscopy. In strong contrast, the broad-band character of the BBC permits an absolutely straightforward execution of 1D and 2D 19 F-NMR experiments. 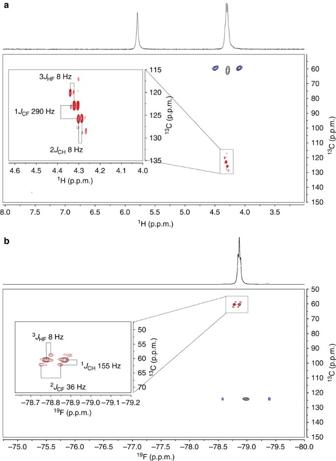Figure 5: Heteronuclear 2D NMR experiments on neat trifluoroethanol. (a)1H13C-HSQC (blue) and1H13C-HMBC (red) reveal1JCH, respectively,1JCF,2JCHand3JHFcoupling constants. (b)19F13C-HSQC (blue) corroborates the relatively large1JCF(the spectral windows are both 2,000 Hz wide); the19F13C-HMBC (red) shows a characteristic skewed doublet-triplet pattern (inset), caused by the1JCH,2JCFand3JHFcoupling constants. Because of the isotope effect, the fluorine resonance signal of a12CF3group is slightly downfield shifted with respect to the averaged resonance signals of13CF3; this is evident from the HSQC cross peaks, and the off-centre CF3triplet signal corresponding with the HMBC cross peak. The HSQC spectra were also acquired in decoupled mode (black). Figure 5 shows spectra of 1 H 13 C-HSQC, 1 H 13 C-HMBC, 19 F 13 C-HSQC and 19 F 13 C-HMBC experiments performed on neat trifluoroethanol, providing detailed information on all the coupling constants in the system. Figure 5: Heteronuclear 2D NMR experiments on neat trifluoroethanol. ( a ) 1 H 13 C-HSQC (blue) and 1 H 13 C-HMBC (red) reveal 1 J CH , respectively, 1 J CF , 2 J CH and 3 J HF coupling constants. ( b ) 19 F 13 C-HSQC (blue) corroborates the relatively large 1 J CF (the spectral windows are both 2,000 Hz wide); the 19 F 13 C-HMBC (red) shows a characteristic skewed doublet-triplet pattern (inset), caused by the 1 J CH , 2 J CF and 3 J HF coupling constants. Because of the isotope effect, the fluorine resonance signal of a 12 CF 3 group is slightly downfield shifted with respect to the averaged resonance signals of 13 CF 3 ; this is evident from the HSQC cross peaks, and the off-centre CF 3 triplet signal corresponding with the HMBC cross peak. The HSQC spectra were also acquired in decoupled mode (black). Full size image Metabolomics NMR spectroscopy is widely applied in metabolomics and analysis of biological fluids in medical diagnostics and drug discovery [33] . To test the performance of our BBC set-up for these purposes, the urinary excretion of taurine was monitored by 1 H-NMR spectroscopy ( Fig. 6 ), revealing its practically quantitative excretion after consumption of energy beverages containing large amounts of taurine. 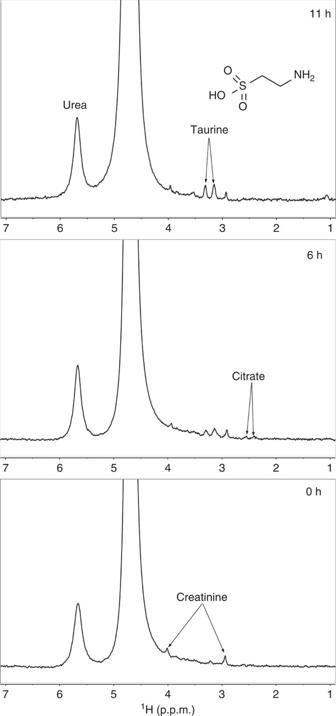Figure 6: 1H-NMR spectra of neat urine. Spectra were taken at different time intervals from a volunteer consuming energy drinks (200 ml h−1for 6 h) containing 0.4% of taurine. The taurine concentrations in the 6 h and 11 h urine samples are about 40 mM, corresponding to a similar taurine concentration in the urine and in the original beverage. Figure 6: 1H-NMR spectra of neat urine. Spectra were taken at different time intervals from a volunteer consuming energy drinks (200 ml h −1 for 6 h) containing 0.4% of taurine. The taurine concentrations in the 6 h and 11 h urine samples are about 40 mM, corresponding to a similar taurine concentration in the urine and in the original beverage. Full size image 19 F-NMR spectroscopy is a particularly useful tool in metabolic analysis, background signals of fluorine being absent in biological systems [32] , [34] . Trifluoromethyl is a functional group present in various medicinal compounds, like the antidepressant fluoxetine (Prozac), and monitoring 19 F blood levels is a powerful tool for determining optimal dosage levels in drug development or for determination of fatal overdoses. Clinically relevant drug concentrations of fluoxetine are in the order of nmol ml −1 ; this first generation BBC set-up can measure down to 25 picomoles, and therefore the amount of drug present in less than 1 ml of blood could be readily detected after a pre-concentration step (for spectra, see Supplementary Fig. 2 ). A front end consisting of a microcoil-on-a-chip terminating a coaxial cable with no tuning and matching circuitry functions as a high-resolution ‘all-in-one’ BBC NMR system, with broad-band character enabling the execution of one- and multidimensional, homo- and heteronuclear, experiments at relatively high fields and with excellent mass sensitivity. Jerschow and co-workers [35] have recently reported on the broad-band capabilities of travelling wave NMR, which concerns an elegantly simple NMR circuit of a conductor connected with a coaxial cable. The proof of principle is promising, but the performance depends strongly on the coaxial cable length and impedance matching and suffers from an inhomogeneous B 1 distribution over the detection sample volume and a rather low sensitivity, limiting a more versatile implementation. The BBC probe is a cheap yet versatile and robust set-up that can detect different nuclides with straightforward applications in on-flow monitoring of chromatographic separations [8] , reactions [16] , and lab-on-a-chip processes [36] , or for further downscaling bacteria and biomarker detection [37] , or intracellular protein identification [38] . Another immediate, noteworthy consequence of the non-resonant concept of the BBC system is that the NMR probe as such is magnetic field-independent, and one and the same probe can be utilized on different (field) NMR systems. Moreover, the small detection volume alleviates the problems related to field homogeneity over large sample volumes and, consequently, BBC probes are likely to play a major role in portable or table-top NMR systems with inhomogeneous magnetic fields or built around compact permanent or cryogen-free superconducting magnets [39] . Besides the direct applications in medical diagnostics, drug or catalyst screening, there are many emerging aspects of this new technology, for dynamic nuclear polarization schemes or for time-saving ‘multinuclear multitasking’ strategies in which acquisition scans are alternated between two kinds of nuclides in a way that while one nuclide is scanned, the other is relaxing. Finally, the possibility to excite and detect simultaneously any number of nuclides (or a superposition of such signals) will lead to the development of new multinuclear pulse sequences and to new application areas. The paradigm shift we present in this paper advocates a thorough re-evaluation of many different aspects of NMR spectroscopy instruments, particularly of the electrical and engineering properties of, for example, coils, circuits and (pre-)amplifiers, which might reveal to be more, or less, relevant in new generation broad-band-coil NMR spectrometers than they are in the current spectrometers utilizing tuned circuits. Materials Chemicals and deuterated solvents were purchased from Sigma-Aldrich and used as received, without further purification. BBC set-up design The microfluidic NMR chips were designed using CleWin Layout Editor version 4.3.3.0 (WieWeb Software, Hengelo, the Netherlands) and fabricated by Micronit Microfluidics BV, Enschede, the Netherlands, using standard microfabrication techniques similar to the ones previously described [40] . The chips have a standard format of 1.5 × 4.5 cm, with rounded V-shaped channels wet-etched 500 μm deep in the bottom of a 1.1 mm thick borosilicate glass wafer. The diameter of the channel is of 500 μm in the detection area and of 250 μm for the rest. Fluidic access holes to these channels were powder blasted also in this wafer. In addition, a larger channel was powder blasted along the smaller wet-etched channel to allow for eventual cooling or heating of the main sample channel. A 100 μm thin glass wafer was used to bond to the channels. For the fabrication of the electrodes and coils, a Cr/Cu seed layer was applied on the backside of this thin glass wafer, and then a 20 μm thick copper layer was applied to create the final structured electrodes. Each planar spiral microcoil consists of 32 turns with a width and separation of 20 μm and an inner diameter of 250 μm (see Supplementary Fig. 1 for details), yielding a total detection volume of 25 nl. The outer turn of the microcoil was directly connected to one of the copper electrode, while the inner turn ending was wire-bonded to the opposite copper electrode. The coil has a low resistance ( ρ =7 Ω) and was directly soldered via bare copper wires to copper transmission lines ending in a BNC connector at the bottom of the probe. Importantly, no tuning or matching capacitors were used in the RF circuit. From the BNC connector, a coaxial cable was connected to the transmitter/receiver channel of the spectrometer. For heteronuclear 2D experiments, a combiner was used to connect the transmitter and decoupler outputs to the single coax cable connected to the BBC set-up. Appropriate high pass or band filters were used in the high-gamma, respectively, low-gamma channels. Details on acquisition parameters are provided in the Supplementary Table 1 . The chip was placed inside a standardized Fluidic Slide that fits into a custom-built aluminium Fluidic Connect chip holder with a diameter of 3.8 cm and a length of 11.2 cm, mounted on top of the aluminium cylinder of a sacrificed (commercial) NMR probe. The chip holder consists of two halves assembled together using brass screws. The front half of the holder was functionalized with microfluidic access holes enabling leak-free connections, while electrical connections to the copper electrodes were accessible from the other half of the holder. The two coils can be addressed contemporaneously or separately, for fast reactions monitoring or for homonuclear or heteronuclear applications, and one of the possibilities is to use one of the coils for a field-lock circuit. The experiments we describe here have been performed using the top coil only. The multiple microfluidic inlets allow for on-chip mixing of reactants or cooling through a separate microfluidic channel. Standard microfluidic connections and plug-and-play electrical connections were purchased from Micronit Microfluidics BV. The geometry and parameters of the proton-tuned microprobe used as control were identical to the non-tuned system, except for the microcoil now being hardwired to the tuning and matching circuit of a standard commercial 400 MHz Varian NMR probe, allowing the tuning and matching of the microcoil circuit using the corresponding rods at the bottom of the probe. An additional variable (3–18 pF) capacitor was added in parallel to the microcoil to allow the resonance circuit to be in the 400 MHz range. NMR experiments NMR experiments were carried out using an Oxford Instruments 9.4 T wide-bore magnet, equipped with a 28-channel shim box, using a Varian INOVA spectrometer. All experiments were acquired in non-locked mode, adjusting shims on the free induction decay. Standard pulse sequences from VnmrJ 2.2D software were used for 1D and 2D experiments, with typical attenuation of transmitter amplifiers of 5 dB. Long acquisition times of the 2D experiments in non-locked mode were not visibly affected by the drift of the magnetic field of less than 1 Hz h −1 . Arrayed experiments were processed with VnmrJ software; the other data were processed using MestReNova 6.2.1 software (Mestrelab Research, Santiago de Compostela, Spain). Control experiments for the heteronuclear 2D limit of detection discussion were performed on a Varian VNMRS-400 NMR system using a 400 ASW PFG (4Nuc/40–162 MHz) probe with standard 5 mm tubes (sample volume of 0.5 ml). The standard VnmrJ PWXCAL pulse sequence, which is normally used to calibrate the pulse width characteristics of the probe’s decoupler channel in indirect detection or triple resonance experiments, was adapted for the indirect calibration of the 90° pulse width of the 13 C channel on a 5 M acetic acid-1- 13 C sample (see Supplementary Fig. 3 ). The delays between the 90 and the 180° pulses were adjusted according to the value of the two-bond proton-carbon coupling constant. The value obtained (20 μs at a transmitter attenuation of 5 dB) was consecutively used in the HSQC and HMBC experiments. For the 1 H 13 C-HSQC and 1 H 13 C-HMBC experiments the standard delays used were calculated from the one-bond ( 1 j CH =140 Hz), respectively, multiple bond ( n j CH =5–6 Hz) proton-carbon coupling constants. For the heteronuclear 19 F 13 C-experiments the corresponding delays were adjusted for the larger one-bond ( 1 j CF =280 Hz) and two-bond ( 2 j CF =36 Hz) carbon–fluorine coupling constants. For the heteronuclear 19 F 31 P experiments the corresponding delays were adjusted for the one-bond ( 1 j PF =710 Hz) phosphorus-fluorine coupling constant. The power level for the transmitter channel (tpwr) was set to 5 dB, and 90° pulses were determined before each experiment and were in the range of 7–11 μs. The acquisition parameters for the heteronuclear 2D experiments described in this article are summarized in the Supplementary Table 1 . Signal-to-noise measurements and mass/molar sensitivity We compared the signal-to-noise ratio on a sample of 25 nl (25 μg, 1.4 μmol) of H 2 O, both in the non-resonant (BBC) and the 1 H-tuned microprobe. A single scan was acquired for each sample at 400 MHz to detect the proton signal with identical acquisition parameters: acquisition time 0.5 s, 1 scan, 2,000 data points. Data were processed with MestReNova, using the same processing parameters for each spectrum: 1 Hz exponential apodization, manual phase correction and full auto baseline correction. The SNR Peak Calculator script in MestReNova was used to determine the signal-to-noise ratio. The obtained values were of 3,165 for the BBC microprobe and 3,185 for the 1 H-tuned microprobe. For mass-limited samples, the mass (molar) sensitivity, S m , is a better figure of merit for comparison of probes with different volumes [8] , and is defined as where m is the molar amount of material in the detection volume and t aq the acquisition time. Therefore, the S m values are of 3220 SNR·μmol −1 s −1/2 for the BBC microprobe and 3,240 for the 1 H-tuned microprobe. Considering the lower magnetic field used in this work (9.4 T, 400 MHz) compared with what is described in literature (14.1 T, 600 MHz), the S m values normalized according to the proportionality factor [B 0 ] 7/4 are 6,546 and 6,587 SNR·μmol −1 s −1/2 , respectively; these values are four times higher than the value of 1,530 SNR·μmol −1 s −1/2 determined for a 620 nl prototype probe from a commercial NMR probe manufacturer [8] . Finite element equivalent-circuit simulations An example of an equivalent-circuit simulation ( Supplementary Fig. 4 ) illustrates the persistent feature of the BBC microcoil. The complex impedance of the coil remains constant and equal to its DC resistance until over 100 MHz when the inductive component starts becoming perceptible. However, the DC impedance continues to be a good approximation of the RF impedance up to at least 500 MHz. Therefore, the coil behaves as a resistive device up and beyond about 100 MHz and for the generation of B 1 , what matters is the current passing along the coil paths (related to the ohmic and inductive components) and not the radial ‘parasitic’ current through the parasitic capacitors. How to cite this article: Fratila, R.M. et al . Multinuclear nanoliter one-dimensional and two-dimensional NMR spectroscopy with a single non-resonant microcoil. Nat. Commun. 5:3025 doi: 10.1038/ncomms4025 (2014).